Klebsormidium flaccidumgenome reveals primary factors for plant terrestrial adaptation The colonization of land by plants was a key event in the evolution of life. Here we report the draft genome sequence of the filamentous terrestrial alga Klebsormidium flaccidum (Division Charophyta, Order Klebsormidiales) to elucidate the early transition step from aquatic algae to land plants. Comparison of the genome sequence with that of other algae and land plants demonstrate that K. flaccidum acquired many genes specific to land plants. We demonstrate that K. flaccidum indeed produces several plant hormones and homologues of some of the signalling intermediates required for hormone actions in higher plants. The K. flaccidum genome also encodes a primitive system to protect against the harmful effects of high-intensity light. The presence of these plant-related systems in K. flaccidum suggests that, during evolution, this alga acquired the fundamental machinery required for adaptation to terrestrial environments. The colonization of land by plants was a key event in the evolution of life, making the modern terrestrial environment habitable by supplying various nutrients [1] and sufficient atmospheric oxygen [2] . It is generally accepted that the ancestor(s) of current terrestrial plants was closely related to present-day charophytes [3] , [4] , [5] . However, the fragmentary genome sequence data available for charophytes has frustrated efforts to find evidence consistent with the proposed transition of a charophyte(s) to the first land plants. The colonization of land by plants must have been preceded by the transition of aquatic algae to terrestrial algae. During this process, the transition species of aquatic algae must have acquired a range of adaptive mechanisms to cope with the harsh features of terrestrial environments, such as drought, high-intensity light and UV radiation [6] . In addition to making these adaptations, land plants needed to simultaneously enlarge their body sizes through cellular differentiation. The primary features that enabled primitive aquatic plants to colonize land have yet to be established. Given that these features must have a genetic basis and that the intermediate genomes of the relatives between aquatic algae and terrestrial plants must lead to clues to these crucial factors, comparative genomic analyses involving charophytic algae—which comprise streptophytes with embryophytes (land plants)—seem critical for elucidation of these features. The charophytic algae Klebsormidium usually consist of multicellular and non-branching filaments without differentiated or specialized cells. Klebsormidium species therefore have primitive body plans, and most species that have adapted to land also can survive in fresh water [4] , [7] . In fact, tolerance to typical terrestrial stresses like drought [8] , [9] , [10] or freezing [9] , [11] has been reported in some Klebsormidium species. These features suggest that an ancestor of modern-day members of Klebsormidiales acquired fundamental mechanisms that enable survival in severe land environments that differ substantially from the more stable conditions characteristic of aquatic environments. Here we sequence and analyse the genome of the K. flaccidum strain NIES-2285 ( Fig. 1 ). Comparison of this genome sequence with available genome sequences of other algae and land plants suggests that K. flaccidum acquired many genes specific to land plants. These include genes essential for plant hormone action and cyclic electron flow (CEF) activity—biological systems that were probably critical for terrestrialization. Our analysis provides evidence that K. flaccidum has the fundamental machinery required for adaptation to survival in terrestrial environments. 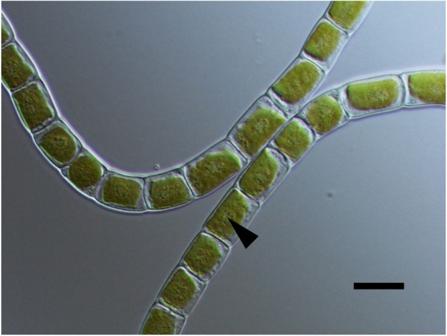Figure 1: Differential interference microscope image ofKlebsormidium flaccidumstrain NIES-2285. K. flaccidumconsists of non-branching long filamentous cells. Each cell contains a large chloroplast, which is positioned against the cell wall (parietal chloroplast) and contains a pyrenoid. Arrowhead indicates a pyrenoid surrounded by a few starch grains. Scale bar, 10 μm. Figure 1: Differential interference microscope image of Klebsormidium flaccidum strain NIES-2285. K. flaccidum consists of non-branching long filamentous cells. Each cell contains a large chloroplast, which is positioned against the cell wall (parietal chloroplast) and contains a pyrenoid. Arrowhead indicates a pyrenoid surrounded by a few starch grains. Scale bar, 10 μm. Full size image Genome sequencing and phylogenetic analysis Total genome size was estimated as 117.1±21.8 Mb ( Supplementary Fig. 1 ), and the DNA and cDNA sequences were determined using both the Roche 454 GS FLX Titanium and Illumina GAIIx platforms ( Supplementary Table 1 ). The sequenced DNA reads were assembled into 1,814 scaffolds covering the nuclear (104 Mb), plastidic (181 kb) and mitochondrial (106 kb) genomes ( Supplementary Table 1 ). We identified and annotated 16,215 protein-coding genes in the nuclear and organellar genomes ( Supplementary Table 1 ). To examine the phylogenetic similarity between K. flaccidum , land plants and other algae, we compared the sequences of 31 highly conserved proteins of 14 species and charophytes ( K. flaccidum , 5 land plants, 7 charophytes algae and 9 other algae; Supplementary Data 1 ). The phylogenetic tree constructed based on the concatenated amino acid sequence alignment of 31 nuclear genes showed that K. flaccidum diverged after Chlorokybus atmophyticus ( Fig. 2 ). This topology was the same as previous reports [3] , [4] , [5] . 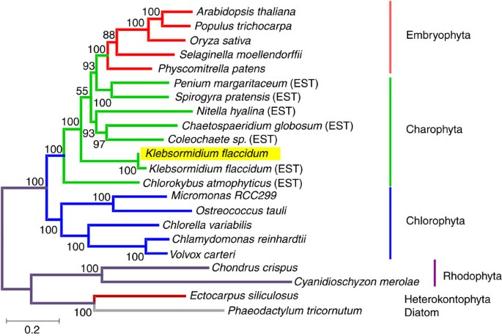Figure 2: Phylogenetic analysis of 31 genes from 21 species of algae and land plants. The phylogenetic tree was constructed as the optimal maximum-likelihood tree with the concatenation of 31 nuclear-encoded protein and translated ESTs (Supplementary Data 1) alignments. Numbers represent support values after 100 bootstrap replicates. The scale bar denotes the number of substitutions per site. Figure 2: Phylogenetic analysis of 31 genes from 21 species of algae and land plants. The phylogenetic tree was constructed as the optimal maximum-likelihood tree with the concatenation of 31 nuclear-encoded protein and translated ESTs ( Supplementary Data 1 ) alignments. Numbers represent support values after 100 bootstrap replicates. The scale bar denotes the number of substitutions per site. Full size image Comparative analyses for gene families and protein domains We classified all proteins from each of the 15 species whose genome sequences were determined ( Fig. 3a and Supplementary Table 2 ), revealing that 1,238 proteins of K. flaccidum are shared by land plants, a number greater than that of other algae, although phylogenetic analysis showed that K. flaccidum is an early diverging lineage of charophytes. Hierarchical clustering ( Fig. 3b ) based on the presence or absence of homologous genes in individual organisms for 5,447 K. flaccidum gene groups commonly found in other species suggested that the K. flaccidum proteins resemble those of land plants more than those of other algae we analysed. The reciprocal best-hit analysis of conserved proteins of both algae and land plants also supported that K. flaccidum has genetic characters similar to those of land plants ( Supplementary Fig. 2 ). 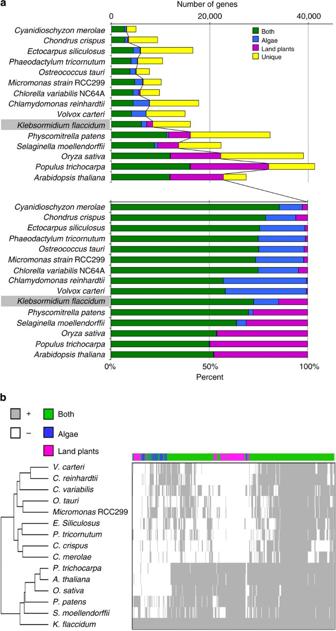Figure 3: Comparison of proteins among 15 species of algae and land plants. (a) Numbers of proteins found in both algae and land plants (green), proteins shared among algae (blue), proteins shared among land plants (magenta), and no reciprocal best hit to other species (yellow) with classification via OrthoMCL (Supplementary Table 2). The upper and lower panels represent the number of genes and the percentage, respectively, for the four categories (the genes without counterparts in yellow were excluded for percentage data). (b) Binary heat map of 5,447 gene groups that were identified as non-unique compared withK. flaccidumand the other 14 organisms studied. The columns and rows represent 5,447 groups ofK.flaccidumand their counterparts from 14 organisms, respectively. Grey shading indicates that the group in the organism includes at least one gene by OrthoMCL analysis; white indicates no orthologous gene. The coloured bar shows the classification of eachK.flaccidumgroups as described fora. Dendrogram on the left corresponds to the results of hierarchical clustering for all organisms. Figure 3: Comparison of proteins among 15 species of algae and land plants. ( a ) Numbers of proteins found in both algae and land plants (green), proteins shared among algae (blue), proteins shared among land plants (magenta), and no reciprocal best hit to other species (yellow) with classification via OrthoMCL ( Supplementary Table 2 ). The upper and lower panels represent the number of genes and the percentage, respectively, for the four categories (the genes without counterparts in yellow were excluded for percentage data). ( b ) Binary heat map of 5,447 gene groups that were identified as non-unique compared with K. flaccidum and the other 14 organisms studied. The columns and rows represent 5,447 groups of K . flaccidum and their counterparts from 14 organisms, respectively. Grey shading indicates that the group in the organism includes at least one gene by OrthoMCL analysis; white indicates no orthologous gene. The coloured bar shows the classification of each K . flaccidum groups as described for a . Dendrogram on the left corresponds to the results of hierarchical clustering for all organisms. Full size image Next, we inferred the history of gene acquisition that enabled terrestrial adaptation by assessing the diversity seen among gene families and protein domains in 15 representative algae and land plants. For this study, paralogues were defined as genes belonging to a gene family containing at least two genes, and singletons were defined as genes lacking any paralogue in each species. The number of gene families was defined as the sum of the gene families of paralogues and singletons ( Supplementary Table 3 ). To represent the diversity within the gene complement of each species, we plotted the number of gene families against the total number of genes ( Fig. 4a ). For algae, the number of gene families increased proportionally with total gene number. This was not the case, however, for land plants owing to an apparent upper limit of the number of gene families. Compared with the algae analysed, the plants studied contained more paralogous genes in each gene family and fewer singletons ( Supplementary Fig. 3 ). For K. flaccidum , we found that many paralogues for which the number in land plants was significantly greater were in fact singletons ( Supplementary Fig. 4 and Supplementary Data 2 ). Notably, these counterpart genes are involved in processes such as cell wall biogenesis, signal transduction, plant hormone-related categories and environmental responses ( Supplementary Data 2 and 3 ). 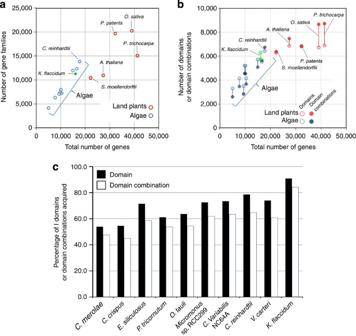Figure 4: Gene families and domains in 15 species of algae and land plants. (a) The green filled circle denotes the data point forK. flaccidum, and red and blue circles denote data points for land plants and algae, respectively (Supplementary Table 3). (b) Number of domains (open circles) and domain combinations (filled circles) expressed in terms of the total number of genes in each of 15 species (Supplementary Table 4). (c) Acquisition in algal genomes of conserved domains (black bars) and domain combinations (white bars) commonly found in land plants. For the land plants analysed (five species), the numbers of conserved domains and domain combinations were 4,894 and 2,801, respectively (Supplementary Table 5). Figure 4: Gene families and domains in 15 species of algae and land plants. ( a ) The green filled circle denotes the data point for K. flaccidum , and red and blue circles denote data points for land plants and algae, respectively ( Supplementary Table 3 ). ( b ) Number of domains (open circles) and domain combinations (filled circles) expressed in terms of the total number of genes in each of 15 species ( Supplementary Table 4 ). ( c ) Acquisition in algal genomes of conserved domains (black bars) and domain combinations (white bars) commonly found in land plants. 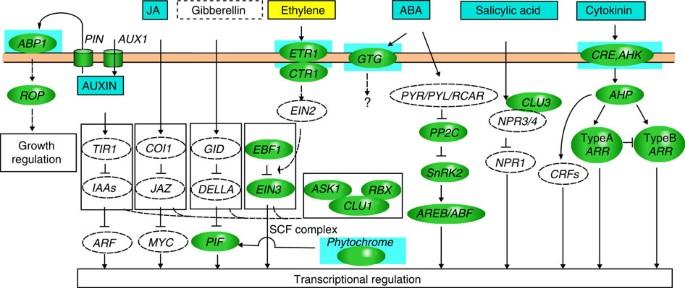Figure 5: Overview of predicted plant hormone signalling inK. flaccidum. Plant hormones were quantified by mass spectrometry (Supplementary Table 6). Boxes highlighted in light blue, yellow, and surrounded by broken lines represent detected, unmeasured, and undetectable plant hormones, respectively. Green ellipses represent putative counterparts, and dashed ellipses represent undetected counterparts (Supplementary Data 5). Receptors for which putative genes were found in theK. flaccidumgenome are indicated against a light-blue background. For the land plants analysed (five species), the numbers of conserved domains and domain combinations were 4,894 and 2,801, respectively ( Supplementary Table 5 ). Full size image In addition to gene families, we also analysed the number of domains and domain combinations, based on the Pfam database [12] , in proteins of the 15 species studied. For domain combinations, the numbers, positions and order of domains in each protein were ignored ( Supplementary Table 4 ). For each species, the number of domains and domain combinations were plotted separately against the total number of genes ( Fig. 4b ). Although the number of domains in each of K. flaccidum , Physcomitrella patens (moss) and Selaginella moellendorffii (spike moss) was the maximal value, for angiosperms (flowering plants) the number of domain combinations continued to increase with increasing gene number. Comparison of the total number of Pfam domains in 15 species revealed that 90.7% (4,441/4,894) of the domains and 84.3% (2,360/2,801) of domain combinations that are commonly found in land plants are represented in the K. flaccidum genome ( Fig. 4c and Supplementary Table 5 ). Thus, many archetypal genes typically found in modern land plants probably had already been acquired by the ancestor of K. flaccidum . During adaptation to the various challenges associated with terrestrial life, the numbers of these genes increased in land plants because additional paralogues were acquired, thereby providing new combinations of domains as a consequence of gene duplication and shuffling in land plants [13] . Streptophyta-specific genes and their roles We next conducted a comprehensive search for systems typically found in land plants that are essential for terrestrial life. The gene ontology categories of the 1,238 Streptophyta-specific genes in K. flaccidum ( Fig. 3a and Supplementary Table 2 ) were assigned based on best hits with respect to Arabidopsis genes/gene families. Several genes are highly enriched in biological process categories such as regulation of transcription, signal transduction, response to various stress conditions, cell wall biogenesis and plant hormone-related functions ( Supplementary Data 4 ). It is reasonable to expect that biological systems involved in these categories contributed to primary terrestrial adaptation. These analyses suggested that an ancestor of K. flaccidum had already acquired genes crucial for terrestrial life. In particular, plant hormone-mediated signal transduction pathways were likely essential for the evolution of responses to environmental stimuli in land plants. Many plant hormones have also been detected in both unicellular and multicellular algae [14] , [15] , but their functions in algae remain mostly unclear. Analysis of the K. flaccidum genome revealed candidates for most of the genes required for the biosynthesis of auxin, abscisic acid (ABA), and jasmonic acid (JA) ( Supplementary Data 5 ). 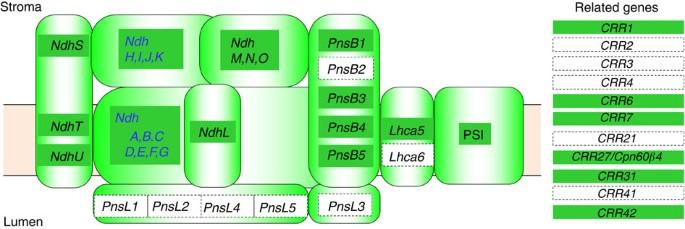Figure 6: Predicted NDH complex and related genes inK. flaccidum. Green boxes indicate that putative counterparts identified, and open boxes surrounded by broken lines indicate that no putative counterparts were found (Supplementary Data 7). Genes with names written in blue reside within the chloroplast genome. Moreover, detection of plant hormones with mass spectrometry unambiguously indicated the presence in K. flaccidum of the auxin indole-3-acetic acid, ABA, the cytokinin isopentenyladenine, JA, and salicylic acid ( Supplementary Table 6 ). In addition, we identified genes predicted to encode counterparts of the plant hormone receptors ABP1 (auxin), GTG (ABA), CRE1 (cytokinin) and ETR (ethylene) ( Fig. 5 and Supplementary Data 5 ). Figure 5: Overview of predicted plant hormone signalling in K. flaccidum. Plant hormones were quantified by mass spectrometry ( Supplementary Table 6 ). Boxes highlighted in light blue, yellow, and surrounded by broken lines represent detected, unmeasured, and undetectable plant hormones, respectively. Green ellipses represent putative counterparts, and dashed ellipses represent undetected counterparts ( Supplementary Data 5 ). Receptors for which putative genes were found in the K. flaccidum genome are indicated against a light-blue background. Full size image We also compared organellar genes found in other algae and land plants. A notable feature of the K. flaccidum plastid genome was the presence of 18 NADH oxidoreductase subunits that constitute the NADH dehydrogenase-like complex (NDH) ( Fig. 6 , Supplementary Data 6 and 7 ), which mediates CEF in photosystemI [16] , [17] , [18] . Several stresses, including high-intensity light and drought, can activate CEF. It is believed that CEF increases the proton gradient across the thylakoid membrane, which induces non-photochemical quenching (NPQ) and ATP synthesis [16] , [19] . These responses dissipate excess light energy and enable various adaptive responses to stress. Land plants have two CEF pathways, namely the PGR5 and NDH pathways [19] , [20] , but no genes encoding NDH have been found in algae except for members of Charophyta and some Prasinophyceae [21] . Here we identified seven genes in the K. flaccidum nuclear genome that encode NDH components and PGR5 ( Supplementary Data 7 ). Although some NDH genes were not identified, the K. flaccidum genome harbours genes that encode major NDH components ( Fig. 6 and Supplementary Data 7 ). A CEF activity mediated by the NDH pathway has been detected as a transient increase in chlorophyll fluorescence after turning off actinic light by pulse-amplitude-modulated fluorometry [22] . Our analysis clearly demonstrated that K. flaccidum has the CEF activity ( Fig. 7a,b ). Figure 6: Predicted NDH complex and related genes in K. flaccidum. Green boxes indicate that putative counterparts identified, and open boxes surrounded by broken lines indicate that no putative counterparts were found ( Supplementary Data 7 ). Genes with names written in blue reside within the chloroplast genome. 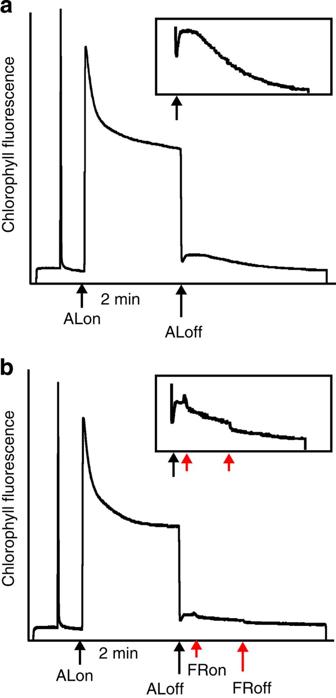Figure 7: Measurement of cyclic electron transport. Transient increases in chlorophyll fluorescence afterK. flaccidumwas kept in the dark (a) or exposed to far-red light (FR, >740 nm,b). Each insert indicates the transient increase in chlorophyll fluorescence after 2 min of illumination with actinic light (AL, 150 μmol m−2s−1). The transient increase of chlorophyll fluorescence in darkness after exposure to actinic light was quenched by subsequent exposure to FR light. These data demonstrate the existence of cyclic electron flow through the NDH pathway. Full size image Figure 7: Measurement of cyclic electron transport. Transient increases in chlorophyll fluorescence after K. flaccidum was kept in the dark ( a ) or exposed to far-red light (FR, >740 nm, b ). Each insert indicates the transient increase in chlorophyll fluorescence after 2 min of illumination with actinic light (AL, 150 μmol m −2 s −1 ). The transient increase of chlorophyll fluorescence in darkness after exposure to actinic light was quenched by subsequent exposure to FR light. These data demonstrate the existence of cyclic electron flow through the NDH pathway. Full size image We showed K. flaccidum produced several plant hormones. Moreover, we found some counterparts for key components in the hormone signalling pathways are encoded in the genome. Of special interest is the likely importance of ABA as a key factor for terrestrialization, because ABA is a central signalling molecule needed to adapt to abiotic stresses such as drought, salinity and freezing [23] . Although we identified counterparts of the hormone receptors ABP1 , GTG , CRE1 and ETR for auxin, ABA, cytokinin and ethylene respectively, we did not detect putative genes for other known receptors, such as TIRs (auxin), PYR/PYL/RCAR (ABA), GID (gibberellin), COI1 (JA-isoleucine) and NPR (salicylic acid) ( Fig. 5 and Supplementary Table 6 ). Among them, the TIRs, GID and COI1 are coupled with protein turnover mediated by the ubiquitin–proteasome system and enable crosstalk among plant hormone signalling pathways [24] , [25] . It is thus interesting that most of the plant hormone signalling machineries that are dependent on SCF (Skp, Cullin and F-box-containing protein) complexes are probably missing in K. flaccidum , although K. flaccidum encodes putative variants of functional receptors and transporters found in land plants, such as ABP1 , PIN [26] and AUX , which are involved in auxin sensing and transport. PINs transport auxin between plants cells and thus have crucial roles in many developmental processes. Arabidopsis produces a novel type of PINs with a short hydrophilic loop in the central region, and these PINs localize to the endoplasmic reticulum [26] . KfPIN was intermediate in size between short- and long-type PINs in our gene models ( Supplementary Figs 5 and 6 ). Further analysis will reveal whether KfPIN directly facilitates auxin transport between cells. Genomic evidence suggests that K. flaccidum has certain types of primitive land-plant signalling pathways for plant hormone responses. The primitive plant hormone responses like those found in K. flaccidum may have further evolved in land plants by coupling with more refined signalling networks such as those involving ubiquitin-mediated proteolysis. These primitive hormone signallings in K. flaccidum may facilitate various responses of this alga to harsh environmental stresses on land. In addition, these hormone systems may play important roles in cell–cell communication in this organism. We tried to find some gene families specific in multicellular organisms ( Clathrus crispus , Ectocarpus siliculosus , Volvox carteri , K. flaccidum and land plants). However, we did not detect any increase in the number of genes that are characteristic of multicellular organisms ( Supplementary Fig. 7 ). In these organisms, multicellularity has evolved independently, and thus comparison between unicellular and multicellular charophytic algae will be necessary to clarify the multicellularity of land plants similarly to study of Volvox [27] . However, genes related to multicellularity ( WUSCHEL , AGAMOUS like MADS-box gene in land plants, GNOM , and several cell wall-related genes) exist in K. flaccidum ( Supplementary Data 5 ). These results suggest that the ancestor of K. flaccidum probably had made a start toward organizing the current complex multicellular systems while it still had a simple body plan. We showed CEF activity in Photosystem I in this alga. Two different inducers of NPQ—PsbS and the Lhc-like polypeptide LHCSR—are known in algae and land plants ( Supplementary Data 7 ). In land plants, NPQ relies mainly on PSBS [28] , whereas in green algae NPQ relies mainly on LHCSR [29] . PSBS and LHCSR work independently through different mechanisms. In P. patens , PSBS and LHCSR act additively to induce strong NPQ for efficient photoprotection [30] . In this regard, K. flaccidum likely relies on LHCSR, whereas PSBS function predominates in the late-diverging charophyta ( Zygnematales , Coleochetales and Charales ) [30] . Although we detected psbS mRNA in K. flaccidum , further work is necessary to clarify the role of PSBS in this alga. Our genome analysis of K. flaccidum reveals the presence and functionality of several important stress responses found in terrestrial plants. Although the protein sets encoded by these genes are primitive, they may be sufficient to guide a primitive body plan and direct the tissue differentiation needed to define a terrestrial alga. Future research on each genomic factor in this organism and further analyses of other charophyte genomes may assist our understanding of the events that enabled plants to colonize land. Genome sequencing and annotation Genomic DNA and expressed mRNAs of K. flaccidum strain NIES-2285 were extracted ( Supplementary Methods ) and sequenced using the Roche 454 GS FLX Titanium and Illumina GAIIx platforms ( Supplementary Methods ). A total of 5.4 Gb (genomic DNA) and 570 Mb (transcriptome) were assembled using Newbler ( Supplementary Methods ). Chloroplast and mitochondrial genomes were assembled independently of the nuclear genome ( Supplementary Methods ). Sequencing and assembly of the nuclear genome was validated using bowtie2, SPALN, BLAST and MEGAN ( Supplementary Methods ). Organellar genes were predicted and annotated using Glimmer3, GeneMarkP, GeneMark (a heuristic approach for gene prediction), FGENESB, tRNAScan-SE, RNAmmer and BLAST with additional manual curation ( Supplementary Methods ). Assembled transcript sequences were mapped to scaffolds using SPALN. Nuclear genes were modelled and predicted by Augustus. These genes were annotated with blast2GO, BLASTP, interpro, Gclust, targetP, ipsort, KAAS, clustalW, MUSCLE, Gblocks and FastTree with additional manual curation ( Supplementary Methods ). The assembled scaffolds sequences have been deposited at DDBJ. The data also can be freely accessed through the project’s website http://www.plantmorphogenesis.bio.titech.ac.jp/~algae_genome_project/klebsormidium/index.html . A basic BLAST tool to search nucleotide and protein databases is accessible at http://genome.microbedb.jp/klebsormidium . Species used for comparative genome analyses K. flaccidum genes were compared with those of nine other algae ( Chondrus crispus [31] , Ectocarpus siliculosus [32] , Phaeodactylum tricornutum [33] , Cyanidioschyzon merolae [34] , Micromonas strain RCC299 (ref. 35 ), Ostreococcus tauri [36] , Chlorella variabilis NC64A [37] , Volvox carteri f. nagariensis [30] , and Chlamydomonas reinhardtii [38] ), eight charophyte ESTs [5] ( Mesostigma viride , Chlorokybus atmophyticus , Klebsormidium flaccidum , Nitella hyalina , Chaetosphaeridium globosum , Coleochaete sp., Spirogyra pratensis , Penium margaritaceum ), and five land plants ( Physcomitrella patens subsp. Patens [6] , Selaginella moellendorffii [39] , Oryza sativa subsp. Japonica [40] , Populus trichocarpa [41] and Arabidopsis thaliana [42] ). Gene data in JGI [43] , Phytozome [44] or the RefSeq [45] release version 54 data set were used for all species except for three algal species— C. merolae , E. siliculosus and C. crispus . These data were used as two data sets: Data set 1 (mainly JGI data) and Data set 2 (mainly refseq data) ( Supplementary Table 7 ). Each data set yielded the same conclusion ( Supplementary Tables 2–5 , Figs 3a,b and 4a–c and Supplementary Figs 3 and 8–12 ). Classification of genes All-against-all BLASTP [46] analysis was applied to all genes of the 15 species analysed ( e -value <1e−3, no filter query sequence). The proteins of each species that were reciprocally assigned the highest scores relative to the genes of the other species were then extracted. Only the proteins of each species for which alignments covered >50% of the query and database sequences were used for this analysis. After extracting the proteins with reciprocal best hits, homologous clusters were identified by clustering analysis using OrthoMCL [47] with following parameters: inflation value=1.5, percentMatchCutoff=1 and evalueExponentCutoff=–3. These homologous clusters were classified into four categories: (1) clusters found only algae, (2) clusters found only in land plants, (3) clusters found in both algae and land plants and (4) no reciprocal best hit to other species ( Fig. 3a , Supplementary Table 2 and Supplementary Fig. 8 ). For this analysis, K. flaccidum was not considered as the reference for both algae and land plants. We also classified homologous clusters into four categories: (1) clusters found only in unicellular organisms, (2) clusters found only in multicellular organisms, (3) clusters found in both unicellular and multicellular organisms and (4) no reciprocal best hit to other species ( Supplementary Fig. 7 ). Heat maps for gene classification First, homologous groups produced by OrthoMCL that contained K. flaccidum genes were selected. As a result, 5,447 gene groups were extracted as non-unique groups shared by K. flaccidum and other organisms and used for subsequent analysis. Against each group, the presence or absence of genes in individual organisms was checked. Then, Pearson’s correlation coefficient between each gene was calculated as a distance matrix, and a gene cluster was constructed using the complete linkage method. Finally, a binary heat map profile with a dendrogram was created ( Fig. 3b and Supplementary Fig. 9 ). All statistical analyses were performed with the R programme version 2.15.1 ( http://www.r-project.org/ ). Phylogenetic tree with Charophyta species A total of 160 ortholog data sets that contained amino acid sequences of Charophyta were obtained from previous research [5] . Sequences originating from Mesostigma were removed from the above data sets because only a few orthologue groups were contained in its EST sequence. BLASTP ( e -value <1e−3, no filter query sequence) was then applied to our K. flaccidum sequence against K. flaccidum sequences within the above data sets to merge the homologous groups produced by OrthoMCL and corresponding Charophyta ortholog groups. In addition, homologous groups for which each algae species had only one sequence were chosen. As a result, 31 homologous groups were selected and merged as the Charophyta ortholog group ( Supplementary Data 1 ). Each merged group was aligned using MAFFT version 6.934 beta [48] with default parameters. Alignments were then concatenated by species. The maximum-likelihood approach was applied to construct a phylogenetic tree using MEGA version 5.05 (ref. 49 ) with the JTT+F+gamma model. In MEGA5, the partial deletion method with an 80% cut off was chosen to remove ambiguous sites ( Fig. 2 ). Reciprocal BLASTP best-hit analysis Statistical analysis of best reciprocal protein and EST hits for K. flaccidum with other organisms was performed as follows. The number of best reciprocal hits for protein or EST pairs for K. flaccidum (16,063 genes) with five plants proteins, nine algae and other seven charophyte algae ESTs were extracted with a BLASTP or TBLASTN-BLASTX [47] reciprocal search ( Supplementary Table 8 and Supplementary Table 9 ). BLASTP bit score analysis of the reciprocal best-hit protein for K. flaccidum between nine algae and five land plants was performed as follows. A total of 5,495 genes in K. flaccidum had reciprocal BLASTP best-hit pairs with both algae and land plant proteins ( Supplementary Data 8 ). These BLASTP and reciprocal BLASTP bit scores with the best-hit proteins of algae and land plants were plotted on the x and y axes, respectively ( Supplementary Fig. 2 ). TBLASTN-BLASTX reciprocal best-hit numbers of Charophyta ESTs to gene families for which the numbers of genes were significantly increased in land plants ( Supplementary Data 2 ) was performed as follows. K. flaccidum protein sequences in each group were used as query sequences. The numbers of reciprocal best hits for K. flaccidum genes in each group were extracted by a TBLASTN-BLASTX reciprocal search with nine charophyte algae EST databases ( Supplementary Table 9 ). In Supplementary Data 5 and Supplementary Data 7 , best candidate counterparts in charophyte ESTs for each K. flaccidum gene were estimated by a TBLASTN-BLASTX reciprocal search with nine charophyte algae EST databases ( Supplementary Table 9 ). Best-hits EST sequences that had sufficient sequence length and an appropriate amino-acid sequence frame for multiple alignment were used to construct a gene phylogenetic tree ( Supplementary Figs 13–73 ). Gene family analysis For this analysis, paralogues were defined as genes attributed to the homologous group of OrthoMCL that contained at least two genes, and the singletons then became the genes lacking a paralogue for each species. Hence, the paralogues and singletons represented a gene family for each species ( Fig. 4a , Supplementary Table 3 and Supplementary Figs 3 and 4 ). Functional estimation of gene families The functions of gene families that belonged to land plants for which the numbers of genes were significantly larger than those of algae (median of land plant gene numbers/median of algal gene numbers ≥10; Supplementary Fig. 4 ) were estimated using A. thaliana GOSLIM data of The Arabidopsis Information Resource ftp site ( ftp://ftp.arabidopsis.org/home/tair/Ontologies/Gene_Ontology/ ). The number of genes in each gene ontology category for A. thaliana proteins in each group was counted, and the top three categories of molecular functions and biological processes are noted in Supplementary Data 2 . The numbers of genes and groups in each gene ontology biological process category are noted in Supplementary Data 3 . Analysis of domains and domain combinations The protein domains of each species were searched with PfamScan [12] using the -pfamB option and Pfam27.0 database. PF13352, PB019699 and PB009748, which are specific to P. patens and highly repetitive, were removed from the analysis. The domains and domain combinations were counted using Perl scripts ( Supplementary Tables 4 and 5 , Fig. 4b,c and Supplementary Figs 11 and 12 ). Functional estimation of Streptophyta-specific genes The 865 A. thaliana counterparts of 1,238 Streptophyta-specific genes ( Fig. 3b ) in K. flaccidum were predicted by BLASTP best hits with the criterion that each best-hit gene be in the same gene family between these two species. The numbers of genes and groups of K. flaccidum for which their Arabidopsis counterparts are found in each gene ontology biological process category were counted using A. thaliana GOSLIM with Perl scripts ( Supplementary Data 4 ). Phylogenetic tree Protein and EST sequences were collected from data set 1 ( Supplementary Table 7 ) and charophyte ESTs ( Supplementary Table 8 ) by BLASTP and BLASTX for phylogenetic analysis of all proteins shown in Figs 5 and 6 and Supplementary Data 5 and 7 . After removing insufficient sequences for phylogenetic analysis (short sequence length, low quality, large deletion, and so on), sequences were aligned with MUSCLE [50] . Gblocks 0.91b [51] was used to remove any poorly conserved regions, and the amino acid substitution model was calculated by Aminosan [52] . Phylogenetic analyses were performed in MEGA-CC ver 5.2 (ref. 53 ) with 500 bootstraps. Bootstrap values higher than 50 are indicated under each branch ( Supplementary Figs 13–73 ). Genes involved in plant hormone biosynthesis and signalling Candidate counterparts in K. flaccidum were estimated by BLAST and phylogenetic analysis ( Supplementary Data 5 ). Supplementary Data 5 also includes information of candidates counterparts in other species. Figure 5 is based on a previous study and reviews [16] , [17] , [54] , [55] , [56] . Multiple alignment, membrane spanning region and hydrophobicity profile of amino acid sequences of PINs were calculated and drawn by MUSCLE [50] , BioEdit [57] , Tmpred [58] and Kyte-Doolittle scale [59] ( Supplementary Figs 5 and 6 ). Plant hormone quantification K. flaccidum cells were statically cultured for 5 days in fresh liquid C medium under continuous light (10 μmol photons m –2 s –1 ). Plant hormones were extracted as described [60] with modifications, as follows. Lyophilized samples (~150 mg) were placed in 14-ml round-bottom tubes and ground into powder with 10-mm ceramic beads and liquid nitrogen with vortexing. The ground samples were extracted with 5 ml of 80% ( v / v ) acetonitrile containing 1% ( v / v ) acetic acid for 1 h with internal standards ( 13 C 6 -JA-isoleucine, d 2 -JA, d 6 -SA, d 6 -ABA, d 2 -IAA, d 2 -GA 1 , d 2 -GA 4 , d 5 -tZ, d 3 -DHZ and d 6 -iP). The supernatants were collected after centrifugation at 1,663 g for 20 min, and the pellets were extracted again with 5 ml of 80% acetonitrile containing 1% acetic acid. The supernatants were collected after centrifugation at 1,663 g for 20 min, and the combined supernatants were further purified for hormone analysis. After removing acetonitrile in the supernatants, the acidic water extracts were loaded onto Oasis HLB cartridge columns (500 mg, 6 ml, Waters, Milford, MA, USA) and washed with 6 ml of water containing 1% ( v / v ) acetic acid to remove highly polar impurities. Fractions containing plant hormones were then eluted with 12 ml of 80% ( v / v ) acetonitrile containing 1% ( v / v ) acetic acid. After removing acetonitrile in the eluate via vacuum centrifugation, the acidic water extracts were loaded onto Oasis MCX cartridge columns (30 mg, 1 ml, Waters). After washing the columns with 1 ml of water containing 1% ( v / v ) acetic acid, acidic and neutral compounds (AN fractions) were eluted with 2 ml of 80% ( v / v ) acetonitrile containing 1% ( v / v ) acetic acid. Ten per cent of each AN fraction was used for SA analysis. After washing the Oasis MCX columns with 1 ml of water containing 5% ( v / v ) ammonia, basic compounds containing tZ, DHZ and iP were eluted with 2 ml of 60% ( v / v ) acetonitrile containing 5% ( v / v ) ammonia. After removing acetonitrile in the remaining 90% of the AN fractions, acidic water extracts were loaded onto Oasis WAX cartridge columns (30 mg, 1 ml, Waters). After washing the columns with 1 ml of water containing 1% ( v / v ) acetic acid, neutral compounds were eluted with 2 ml of 80% ( v / v ) acetonitrile and fractions containing acidic compounds (IAA, ABA, JA, JA-isoleucine, GA 1 and GA 4 ) were collected with 2 ml of 80% ( v / v ) acetonitrile containing 1% ( v / v ) acetic acid. Hormones were quantified with liquid chromatography-coupled electrospray ionization–tandem mass spectrometry. The LC gradient condition of ABA, GA 1 , GA 4 ,IAA, JA and JA-Ile was as follows: Solvent A (water containing 0.01% acetic acid), Solvent B (acetonitrile, 0.05% acetic acid) The gradients were programmed for changes of 3–50% composition of solvent B over 15 min [60] . The LC gradient condition of SA was as follows: Solvent A (water containing 0.1% formic acid) and Solvent B (acetonitrile, 0.1% formic acid). The gradients were programmed for changes of 3–98% composition of solvent B over 10 min [60] . The LC gradient condition of tZ, DHZ and iP was as follows: Solvent A (water containing 0.01% acetic acid) and Solvent B (acetonitrile, 0.05% acetic acid) The gradients were programmed for changes of 3–22% composition of solvent B over 27 min [60] . Detected plant hormones were summarized in Supplementary Table 6 . Genes involved in cyclic electron transport Ndh genes in chloroplast genomes of 198 species were listed in Supplementary Data 6 . Candidate counterparts in K. flaccidum were estimated by BLAST and phylogenetic analysis ( Supplementary Data 7 ). Supplementary Data 7 also includes information of candidate counterparts in other species. Figure 6 is based on the composition of the NDH complex determined for land plants [22] . Measurement of cyclic electron transport Cells of K. flaccidum were spotted onto a Protran nitrocellulose membrane (Whatman, Dassel, Germany) by vacuum filtration and adapted to darkness by incubation in the dark for 5 min. CEF of the spotted cells was monitored by MINI-PAM (Waltz, Effeltrich, Germany). Cells were exposed to actinic light (150 μmol m –2 s –1 ) for 2 min. Far-red light was generated by filtering halogen light through a Fuji SC74 filter (>740 nm). The transient increase of chlorophyll fluorescence in the presence or absence of far-red light was then compared ( Fig. 7a,b ). Other analysis Methods for organellar genomes assembly ( Supplementary Fig. 74 ), nuclear genome validation ( Supplementary Figs 75–77 ), organellar genes ( Supplementary Fig. 78 , Supplementary Tables 10 and 11 ), transposable elements prediction ( Supplementary Tables 1 and 12 ), non-coding RNAs prediction ( Supplementary Tables 1 and 12 ) and genome duplication ( Supplementary Figs 79 and 80 ) are described in Supplementary Methods . Accession codes : The assembled nuclear, plastidic, and mitochondrial genome sequences of K. flaccidum , strain NIES-2285, have been deposited in DDBJ/EMBL/GenBank under the accession codes DF236950 to DF238763 ; BioProject ID PRJDB718 . How to cite this article: Hori, K. et al. Klebsormidium flaccidum genome reveals primary factors for plant terrestrial adaptation. Nat. Commun. 5:3978 doi: 10.1038/ncomms4978 (2014).